Dynamic spin polarization by orientation-dependent separation in a ferromagnet–semiconductor hybrid Integration of magnetism into semiconductor electronics would facilitate an all-in-one-chip computer. Ferromagnet/bulk semiconductor hybrids have been, so far, mainly considered as key devices to read out the ferromagnetism by means of spin injection. Here we demonstrate that a Mn-based ferromagnetic layer acts as an orientation-dependent separator for carrier spins confined in a semiconductor quantum well that is set apart from the ferromagnet by a barrier only a few nanometers thick. By this spin-separation effect, a non-equilibrium electron-spin polarization is accumulated in the quantum well due to spin-dependent electron transfer to the ferromagnet. The significant advance of this hybrid design is that the excellent optical properties of the quantum well are maintained. This opens up the possibility of optical readout of the ferromagnet's magnetization and control of the non-equilibrium spin polarization in non-magnetic quantum wells. The unique properties of semiconductors (SCs), which can be adjusted almost arbitrarily according to specific demands, have revolutionized the fields of electronics and optoelectronics. On the basis of this success, it appeared highly attractive to seek strategies to tailor the magnetic properties of SCs as well. An integration of magnetism into SC electronics, for example, would facilitate an all-in-one-chip computer. The goal that has to be targeted in that respect is a ferromagnetic semiconductor, combining the high mobility of charge carriers in SCs and the magnetism of conventional ferromagnets (FMs). This vision has triggered intense activities in which, from the start, the most direct strategies towards this goal have been pursued. Remarkable progress has been made to date, but considerable problems still need to be overcome, calling for elaborate solutions. Most straightforward is the concept of fabricating SCs where the whole functional area is inherently ferromagnetic. So far, however, low-temperature FM semiconductors (such as GaMnAs, InMnAs) show rather poor mobility [1] for charge-carrier transport. Currently, it seems difficult to fulfil the several demanding requirements for a monolithic semiconductor structure with ferromagnetic properties. This underlines the necessity to seek novel concepts, in which the FM layer has a more 'passive', indirect role. Alternative strategies have been envisioned that can be described as hybrid ferromagnet–semiconductor (FM–SC) systems, in which the different constituents take over the separate tasks required for making the device functional as a whole [2] . Examples are direct spin injection devices [3] , [4] , where spin-oriented carriers are injected from the FM, having still an active role, into the SC [5] . Spin polarization could be obtained in that way with an efficiency of up to a few tens of percent [6] , but challenges remain such as the quite high electrical resistance mismatch, the control of the FM's magnetization, and so on. In such a FM–SC hybrid system, each component has to retain its basic properties without deteriorating the properties of the other component: the semiconductor preserves high charge carrier mobility, and the ferromagnet maintains its magnetic properties up to room temperature. Selection of an optimal FM–SC combination out of a great number of possible material combinations is the key challenge here. An indispensable condition for integration, besides readout of the FM, is electrical control of the FM by means of the SC [2] . Towards this goal, one might think about spin-transfer torque control by a high density (~10 8 A cm −2 ) electric current [7] , [8] , [9] , similar to metallic systems. However, such a huge current density would damage the semiconductor. The threshold is decreased down to 10 5 A cm −2 in the low-temperature Mn-based ferromagnetic semiconductors [10] . Another approach is related to multiferroics [11] —electric field effect devices combining magnetic order and ferroelectricity. It remains to be seen whether the implementation of multiferroics into semiconductor electronics is feasible. Alternatively, the application of an electric field has been suggested (the magnetopiezoelectric effect) [12] for switching the magnetization orientation in the FM–SC hybrid. Ref. 13 proposed a structure comprising a FM near a SC quantum well (QW) with a two-dimensional hole gas. The p - d exchange interaction of the magnetic atoms with the QW holes induces an equilibrium spin polarization of the holes, which, in turn, influences the orientation of the magnetization M . The unified FM–SC spin system is highly flexible, as it is possible to control the magnetic anisotropy both optically and electrically. The creation of a flexible FM–SC system comprises the spin polarization of carriers in the QW and the FM control through the spin-polarized charge carriers. Today, researchers have addressed only the first step: spin polarization of charge carriers within a SC quantum well, owing to the interaction with a Mn-based FM, was evidenced by the circularly polarized photoluminescence (PL) [14] , [15] . This observation was interpreted as equilibrium polarization of the hole spins in the exchange field of the Mn spins, in accordance with the predictions of ref. 13 . Here we propose a novel concept of spin polarization in a QW, which can be termed as selective spin separation. It aims to induce spin polarization of SC electrons as well as to read the ferromagnetism in the FM/QW hybrid. The FM is placed a few nanometers apart from a semiconductor QW and serves as a spin selective extractor of QW electrons. By choosing a separation of 5–10 nm, the excellent optical quality of the QW is maintained. Photo-excited QW electrons, with spins either along or opposite to the magnetization of the ferromagnetic layer, are captured by the FM at different rates. This leads to accumulation of electron-spin polarization in the QW, resulting in a circular polarization of the PL. The magnetic hysteresis loop of the FM layer can be traced from both the PL polarization and the PL intensity, which opens possibilities for optical reading of the ferromagnetism and control of the non-equilibrium electron spin through the neighbouring FM. The s(p)-d exchange interaction between FM and QW spin carriers across the separation layer is suppressed. The spin-separation effect is not restricted to optical injection, but must be taken into account also for electrical injection of electrons. Spin orientation of photoexcited carriers by FM layer The experiments were carried out on GaAs-based structures ( Fig. 1a ) with a Mn δ -layer separated from the 10-nm wide InGaAs QW (about 10% of In content) by a 2, 5 or 10-nm thick spacer. The samples are labelled according to this spacer thickness, d s , '2 nm', '5 nm' and '10 nm', respectively. Because of diffusion of Mn ions, the δ -layer is transformed into an ~1-nm thick ferromagnetic layer of Ga 1−x Mn x As with a Mn content x~5% (ref. 16 ). The structural analysis in ref. 16 confirmed the absence of Mn atoms inside the QW. The Mn ions supply holes with a density ~10 13 –10 14 cm −2 , mediating the ferromagnetism of the GaMnAs layer with a Curie temperature T c ~35 K. A relatively small fraction of the holes with concentration ~10 11 cm −2 may populate the QW. A detailed description of the samples is given in ref. 17 . Below, we shall mainly focus on the '10 nm' sample, in which the spin separation occurs and is evidenced through the intense PL under QW resonant optical excitation. 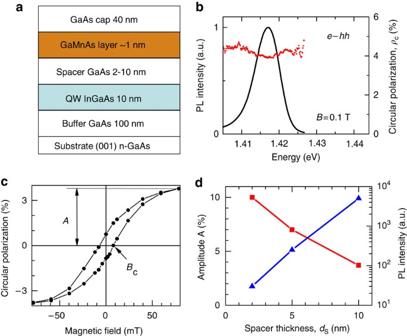Figure 1: Spin orientation of photoexcited carriers by FM layer. (a) Scheme of structures. (b) Spectra of photoluminescence (PL) intensity (black curve) and polarization (red points) for '10 nm' sample under linearly polarized excitation with photon energy 1.92 eV and power 2 mW. (c) Polarization hysteresis loopρc(B) in Faraday geometry in '10 nm' sample for the transitione–hh;Bcis the coercive force;A≡ρc(80 mT). (d) Dependence of amplitudeA(squares) and PL intensity (triangles) on the spacer thickness. TemperatureT=2 K. Figure 1: Spin orientation of photoexcited carriers by FM layer. ( a ) Scheme of structures. ( b ) Spectra of photoluminescence (PL) intensity (black curve) and polarization (red points) for '10 nm' sample under linearly polarized excitation with photon energy 1.92 eV and power 2 mW. ( c ) Polarization hysteresis loop ρ c ( B ) in Faraday geometry in '10 nm' sample for the transition e–hh ; B c is the coercive force; A ≡ ρ c (80 mT). ( d ) Dependence of amplitude A (squares) and PL intensity (triangles) on the spacer thickness. Temperature T =2 K. Full size image For laser illumination with photon energy, =1.92 eV, exceeding the energy gap of the GaAs barrier , the PL spectrum consists of emission from the QW with a maximum at about 1.417 eV ( Fig. 1b ). This emission arises from recombination of electrons and heavy holes ( e–hh ) in their QW ground states. There are also two lines from the GaAs buffer layer (not shown), corresponding to the band-shallow acceptor transitions (1.49 eV) and the exciton – impurity complex recombinations (1.51 eV). The contact with the nearby ferromagnet induces a spin polarization of charge carriers in the non-magnetic semiconductor owing to interaction with the FM's spins [18] , [19] . This spin polarization can be detected from the degree of PL circular polarization ( I ± are the intensities of the σ ± -polarized PL components). In Fig. 1b, the red points show the spectral dependence of ρ c in an external magnetic field B of 0.1 T strength in Faraday geometry ( B || [001]). The e–hh transition in direct vicinity of the FM layer is clearly polarized (in the structures without Mn in such weak magnetic fields, PL polarization is absent). At the same time, the electrons in the GaAs buffer (optical transitions at 1.49 and 1.51 eV) are not polarized. Thus, the transfer of electron spin from the FM into the SC bulk [20] is negligible in such a structure, so that the detection of ferromagnetism is local (<10 nm resolution). Figure 1c shows the polarization hysteresis loop ρ c ( B ), measured at the PL maximum under linearly polarized above-barrier excitation ( =1.54 eV, excitation density 20 W cm −2 ). The coercive force is determined to be B c ~9 mT, and the polarization A ≡ ρ c (80 mT), measured at 80 mT field strength (when the loop becomes closed), is 3.5 %. The appearance of hysteresis demonstrates that the polarization degree of QW emission is controlled by the GaMnAs FM layer (magneto-optical Kerr rotation reveals a hysteresis loop with a shape that is similar to the one in Fig. 1c ). The magnetization of this layer is, however, detected by carriers localized in the InGaAs QW. The presence of hysteresis also means that the easy axis of magnetization is non-orthogonal to the growth axis [001], as reported for GaAs/AlGaAs structures with a δ –Mn layer [14] . Fundamental for this work are two questions: which charge carriers in QW detect the FM, and what is the origin of their spin orientation? At first sight, one may assume that an equilibrium spin polarization of SC charge carriers is established by the effective magnetic field due to the s(p)-d exchange interaction of the carriers with Mn-ions [13] , [14] , [15] . The degree ρ c is determined by the spin polarizations of electrons and/or holes, which, in turn, are proportional to the magnetization M ( B ) of FM. The sign of ρ c is positive at B =+80 mT. In the GaMnAs layer the equilibrium Mn spin with a g -factor of g =+2 is directed against the external magnetic field B . Therefore, the equilibrium spin of QW holes (QW electrons) would be oriented along (against) the magnetic field, because of the antiferromagnetic (ferromagnetic) [21] p - d ( s - d ) coupling with Mn spins. According to the selection rules, the contribution of both charge carriers to the PL polarization would have to be positive, as observed experimentally. However, the experiments presented in the following do not support the explanation based on an equilibrium spin polarization. The blue triangles in Fig. 1d show a considerable drop of the PL intensity (note the logarithmic scale of the right axis) as the spacer thickness decreases. This hints at an effective capture of charge carriers by the FM owing to tunnelling through the GaAs spacer. The red squares in Fig. 1d (left axis) show the dependence of the polarization A on d s , which is nearly linear. In contrast to it, the equilibrium spin polarization model due to s(p)-d exchange predicts an exponentially steep d s -dependence (analogous to the PL intensity dependence) for the exchange coupling strength and, consequently, also for the equilibrium spin polarization, much stronger than found in experiment. Electron spin-separation effect The pronounced spectral dependence of intensity and polarization of the QW PL on the excitation intensity indicates that the PL polarization ρ c is determined by a non-equilibrium spin polarization of electrons, that is, the effect is a dynamic one [22] . For low excitation power (2 mW), the PL line possesses minimum width, and ρ c ( B =0.1 T) varies only slightly across the spectral line ( Fig. 1b ). Under strong excitation power (43 mW), however, the photoexcited carriers fill up the QW, so that the PL line broadens ( Fig. 2a ). This effect is not related with lattice heating because the PL spectrum does not change when the temperature is increased up to the Curie temperature. Simultaneously, we observe a strong spectral dependence of ρ c ( Fig. 2a ): at the low-energy flank, ρ c is about 1%, but at the high-energy side, ρ c is strongly increased to 4%. This behaviour is in accord with the energy diagram in Fig. 2b . QW electrons retain their spin polarization acquired from the interaction with the FM. As a result, the Fermi levels and for spin-up and spin-down electrons are different, leading to an increase of spin polarization on the high-energy side of PL spectrum [23] . At the band bottom, the electron polarization is weaker, and, therefore, ρ c at the low-energy side is reduced. Holes with momentum projections +3/2 and –3/2 onto the growth axis have the same quasi-Fermi level μ h due to their fast spin relaxation (see the next subsection). The polarization degree in Fig. 2a should be inspected for energies above 1.41 eV to eliminate the influence of the superimposed transition showing up as a small shoulder with energy close to the recombination energy of an electron with a Mn acceptor impurity in bulk GaAs [21] . This shoulder may arise from resonant excitation of the GaAs cap layer but does not come from the QW. This transition is beyond the scope of this paper. 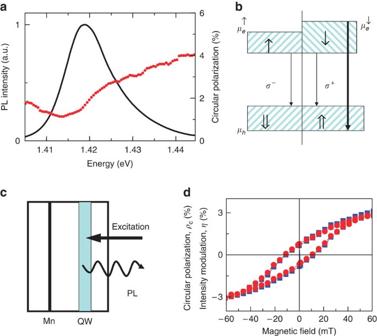Figure 2: Demonstration of electron-spin separation in '10 nm' sample. (a) Spectra of photoluminescence (PL) intensity (black) and PL polarization (red) in a fieldB=0.1 T under excitation by linearly polarized light with=1.92 eV and power 43 mW. (b) Scheme of optical transitions for QW occupied with carriers.andμhare the Fermi levels of electrons with spin up (down) and holes, respectively. (c) Geometry of experiment. Excitation and detection are carried out through the substrate to eliminate the magnetic circular dichroism effect in FM layer. (d) Comparison of the magnetic hysteresis measured in Faraday geometry by PL circular polarizationρc(red circles) and by PL intensity modulationη(blue squares). TemperatureT=2 K. Figure 2: Demonstration of electron-spin separation in '10 nm' sample. ( a ) Spectra of photoluminescence (PL) intensity (black) and PL polarization (red) in a field B =0.1 T under excitation by linearly polarized light with =1.92 eV and power 43 mW. ( b ) Scheme of optical transitions for QW occupied with carriers. and μ h are the Fermi levels of electrons with spin up (down) and holes, respectively. ( c ) Geometry of experiment. Excitation and detection are carried out through the substrate to eliminate the magnetic circular dichroism effect in FM layer. ( d ) Comparison of the magnetic hysteresis measured in Faraday geometry by PL circular polarization ρ c (red circles) and by PL intensity modulation η (blue squares). Temperature T =2 K. Full size image The above experiments point towards a dynamic effect, in which electrons acquire a non-equilibrium spin polarization that is proportional to M . Earlier, the non-equilibrium polarization of free electrons in MnAs/bulk-GaAs structures [20] was explained [24] by their spin-dependent reflection from the FM/SC heterointerface. However, in our case spin polarization is induced even for below-barrier excitation ( ), for which carriers are excited in the QW only. Therefore, one should rather interpret the data in terms of a spin-dependent capture (SDC) of electrons by the FM, which is most efficient if its characteristic rate exceeds the rate of radiative recombination of electrons with holes in the QW. An efficient carrier capture is also indicated by the drastic decrease of PL intensity (and the PL decay time [17] ) for decreasing spacer thickness ( Fig. 1d ). The SDC results in an accumulation of electrons with spin opposite to those leaving the QW faster. This effect is not related to the equilibrium spin polarization in the exchange field of the FM, but is rather a non-equilibrium orientation of electrons, in which the SDC by the FM has the role of a spin separator. Symmetry arguments suggest that the SDC rates γ + ( γ − ) should be different for electrons with spins along (against) the magnetization. An important consequence of SDC must be the dependence of the total PL intensity from the QW on the helicity of exciting light, which generates electrons with spin oriented along or against the magnetization M . The experiment schematically shown in Fig. 2c confirms this hypothesis. Figure 2d compares the magnetic hysteresis measured on '10 nm' sample through ρ c (the red circles) and the parameter (the blue squares), which characterizes the difference in PL intensity between I σ + and I σ − as the helicity of exciting light changes from σ + to σ − . In the first case, a linearly polarized laser excites the QW, and ρ c is measured (a photoelastic modulator is implemented in the PL-detection pathway). In the second case, the circular polarization of the exciting light (the photoelastic modulator is now placed in the excitation pathway) is modulated, and there is a depolarizing wedge in the detector path. To eliminate the effects of magnetic circular dichroism in the GaMnAs layer, we excited the QW through the substrate side, which is transparent for photons with energy =1.44eV. The sizable PL intensity modulation of η ~3% is a clear signature of the SDC. Surprisingly, the dependences ρ c ( B ) and η ( B ) in Fig. 2d coincide, indicating that both quantities are closely related to each other (excitation and detection through the FM gives <0.5% difference due to the magnetic circular-dichroism contribution). Indeed, theoretical consideration of the optical orientation of QW electrons ( Supplementary Methods ) shows that in case of SDC the remarkable relation holds. Here P i is the initial polarization of the electrons excited in the QW by circularly polarized light. This expression is valid for any ratio of the times of radiative recombination τ , of spin relaxation τ S , and of electron capture γ −1 by the FM (the mean capture rate γ =( γ + + γ − )/2). For resonant excitation of the QW heavy-hole subband, the value of P i is close to unity so that the magnetic field dependences of ρ c ( B ) and η ( B ) coincide, in accordance with experiment. Effect of the ferromagnet on optical orientation of QW electrons The Hanle effect [25] of optically oriented QW electrons, in a magnetic field B applied along the well plane (Voigt geometry), enables one to detect the ferromagnetism through the spin precession about the magnetic fields B ex generated by the FM. These measurements therefore allow us to estimate the electron-spin splitting Δ E ex due to the interaction with the FM. The splitting Δ E ex originates mainly from the exchange interaction with the FM and the hyperfine interaction with dynamically polarized nuclei ( Supplementary Discussion ). Circularly polarized continuous wave (cw) excitation injects electron spins polarized along the growth axis [001]. In turn, the electron-spin polarization is registered by the degree of circular PL polarization. The magnetic field in Voigt geometry induces electron-spin precession and PL depolarization, that is, the Hanle effect. To exclude dynamic nuclear polarization by optically oriented electrons, the helicity of the excitation was modulated with a photoelastic modulator at 40 kHz. 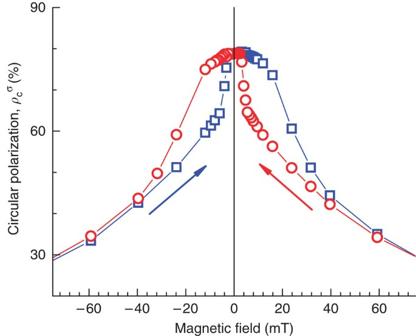Figure 3: Hanle effect of optically oriented QW electrons in '10 nm' sample. Red circles (blue squares) are measured for decreasing (increasing) magnetic field. The dependence(B|| [110]) was measured for QW excitation by light with circular polarization modulated at 40 kHz frequency (). TemperatureT=2 K. Figure 3 shows that an in-plane magnetic field of 30 mT (loop is closed, FM is magnetized) depolarizes the PL by a factor of 2, so that the maximum value of the field B ex cannot exceed the Hanle curve half-width of B 1/2 ~≈30 mT. Thus, the splitting is (for an electron g -factor of | g e | =0.53). This is more than 8,000 times less than the estimated 8.5 meV spin splitting of an electron inside Ga 1−x Mn x As with x=0.05 and s-d exchange constant of 170 meV (ref. 26 ). Figure 3: Hanle effect of optically oriented QW electrons in '10 nm' sample. Red circles (blue squares) are measured for decreasing (increasing) magnetic field. The dependence ( B || [110]) was measured for QW excitation by light with circular polarization modulated at 40 kHz frequency ( ). Temperature T =2 K. Full size image Another way to estimate the splitting Δ E ex follows from time-resolved pump-probe Kerr rotation experiments. Time-resolved pump-probe Kerr rotation traces the electron and hole-spin precession and relaxation [27] , [28] . Typical Kerr rotation signals for different transverse magnetic fields, applied to the '10 nm' sample at T =8 K, are shown in Fig. 4 . The oscillations result from the electron-spin precession with Larmor frequency Ω L about the sum of external field and the field due to the interaction with the FM. The fast decay is attributed to the spin relaxation of holes with τ S h = 20 ps. The long decay time T S = 0.3 ns describes the lifetime of optical orientation. The inverse electron-spin lifetime 1/ T S = 1/ τ S + Γ , where Γ −1 is the electron lifetime and τ S is the electron-spin-relaxation time. Under application of an external magnetic field B , the long-living component oscillates with the Larmor frequency Ω L = | g e | μ B B /ħ and can be described well by the form cos(Ω L t )exp(− t / T S ). The linear dependence of Ω L ( B ) does not go through the zero point (inset in Fig. 4 ). The crossing point with the y axis gives an estimate of the Δ E ex = 2.4 μeV. This value is in good agreement with the estimations from the cw Hanle effect measurements. The equilibrium spin orientation due to this splitting is (k B is a Boltzmann constant), at temperature T =8 K, and cannot explain the much more strongly polarized PL signals with 5% polarization ( Fig. 1c ). Hence, the equilibrium polarization of electrons is negligible in the studied sample. The equilibrium spin polarization of photoexcited holes is also negligible but for another reason: the short spin-relaxation time of holes is not seen in the spin-separation kinetics. 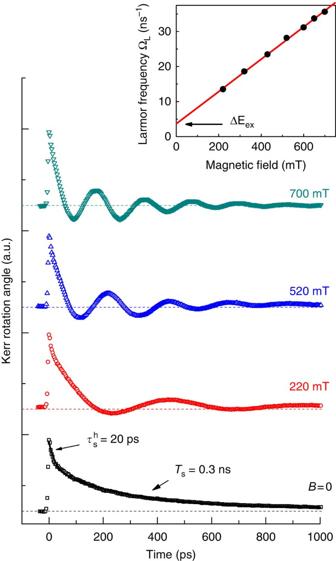Figure 4: Time-resolved Kerr-rotation. Kerr rotation signals as function of delay between pump and probe pulses for different transverse magnetic fields (Voigt geometry). The data are taken at temperatureT=8 K in '10 nm' sample. The curves are shifted vertically for clarity. The solid line for zero field (B=0) data is a fit using a double exponential decay. Inset shows the magnetic-field dependence of Larmor frequency. A linear fit gives |ge| =0.53, corresponding to electrong-factor. The crossing with theyaxis gives an estimate of the splitting of electron ΔEex=2.4 μeV owing to interaction with FM layer. Figure 4: Time-resolved Kerr-rotation. Kerr rotation signals as function of delay between pump and probe pulses for different transverse magnetic fields (Voigt geometry). The data are taken at temperature T =8 K in '10 nm' sample. The curves are shifted vertically for clarity. The solid line for zero field ( B =0) data is a fit using a double exponential decay. Inset shows the magnetic-field dependence of Larmor frequency. A linear fit gives | g e | =0.53, corresponding to electron g -factor. The crossing with the y axis gives an estimate of the splitting of electron Δ E ex =2.4 μeV owing to interaction with FM layer. Full size image Kinetics of the spin-separation effect Time-resolved PL allows one to monitor directly the accumulation of electron spins in the QW and to obtain dynamical parameters of this process: the PL decay rate , the spin relaxation time τ S , and the difference γ + − γ − between the SDC rates. The results are summarized in Fig. 5 . From Fig. 5a, it follows that the PL intensity decays exponentially with a time constant Γ −1 =0.4 ns (in reasonable agreement with the pump probe data in Fig. 4 with T S =0.3 ns). The time evolutions of the circular polarization ρ c and of the modulation parameter η are shown in Fig. 5b . At the time of pulse arrival t =0, both quantities are zero, as there is no equilibrium spin polarization in the QW. Both parameters follow then the same linear increase in time, and change their sign when the external magnetic field is reversed. From a linear fit to the data, we obtain ( γ + − γ − ) −1 =5.5 ns, which is much longer than the electron lifetime and hence the linear approximation holds. In this case of pulsed excitation, the remarkable relation of equation (1) between ρ c ( B ) and η ( B ) also holds, similar to the regime with continuous wave excitation ( Supplementary Methods ). The time dependence of the PL polarization under circularly polarized excitation is shown in Fig. 5c . Initially, within the first 20 ps, there is a fast decay attributed to spin relaxation of the holes. It is not seen in the spin-separation dynamics in Fig. 5b . Hence, we can exclude the hole contribution to the spin-separation effect. The long decay with τ S = 9 ns at B =0 is due to the electrons. The electron-spin relaxation time increases up to 30 ns for application of an external field with 125 mT strength. Such a field converts the multi-domain FM into a single magnetic domain. It leads to the suppression of the QW electron-spin dephasing owing to the coupling with FM domains. The spin relaxation time decreases with temperature (down to 1 ns at 20 K) and therefore the Dyakonov–Perel' mechanism [25] starts to dominate. 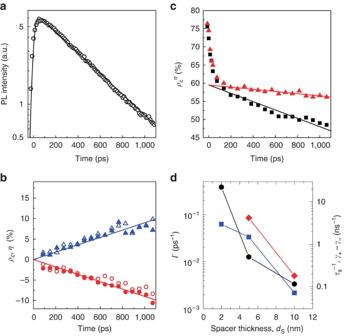Figure 5: Kinetics of spin-separation effect. (a–c) Time-resolved data for '10 nm' sample. (a) Photoluminescence (PL) intensity transient (dots) fitted with an exponential decay convoluted with the apparatus function (line).Γ−1=0.4 ns. (b) Appearance of circular polarizationρc(full symbols) under linearly polarized excitation and modulation parameterη(empty symbols) forB=+125 (triangles) and −125 mT (circles). (c)decay under circular polarized excitation forB=0 (black) andB=125 mT (red). In this case, the average ofmeasured for opposite field directions corresponds to the optical orientation signal. This allows us to exclude odd-B effects related to SDC. Lines in (b) and (c) are linear fits to the data. (d) Dependence of the dynamical parameters on spacer thickness: PL decay rateΓ(squares), difference between the SDC ratesγ+–γ–(diamonds), and electron-spin relaxation rate 1/τS(circles). TemperatureT=2 K. Figure 5: Kinetics of spin-separation effect. ( a – c ) Time-resolved data for '10 nm' sample. ( a ) Photoluminescence (PL) intensity transient (dots) fitted with an exponential decay convoluted with the apparatus function (line). Γ −1 =0.4 ns. ( b ) Appearance of circular polarization ρ c (full symbols) under linearly polarized excitation and modulation parameter η (empty symbols) for B =+125 (triangles) and −125 mT (circles). ( c ) decay under circular polarized excitation for B =0 (black) and B =125 mT (red). In this case, the average of measured for opposite field directions corresponds to the optical orientation signal. This allows us to exclude odd-B effects related to SDC. Lines in ( b ) and ( c ) are linear fits to the data. ( d ) Dependence of the dynamical parameters on spacer thickness: PL decay rate Γ (squares), difference between the SDC rates γ + – γ – (diamonds), and electron-spin relaxation rate 1/ τ S (circles). Temperature T =2 K. Full size image The dynamical parameters and their dependence on the spacer thickness are shown in Fig. 5d . Here in addition to time-resolved photoluminescence, we used time-resolved pump-probe technique with 2 ps time resolution to measure the decay rate Γ in the '2 nm' sample. It follows that Γ varies exponentially steep with d s , which hints at the strong contribution of electron capture by the FM layer. In agreement with that, the SDC rate γ + − γ − amounts to 4 ns −1 for d s =5 nm, which is 25 times larger as compared with the '10 nm' sample. The spin relaxation time decreases significantly with reducing spacer thickness, being about 2 ns and 45 ps for the samples with d s =5 and 2 nm, respectively. However, the relative capture rate difference determining the steady-state polarization varies smoothly with d s , in agreement with Fig. 1d . We come to the conclusion that the spin polarization in these structures has a non-equilibrium, dynamic character. Most likely, the spin imbalance in the density of states in the FM and/or spin-dependent tunnelling is responsible for the capture process. An equilibrium orientation of the charge-carrier spins is practically absent. The spin-separation effect disappears above the Curie temperature of about 35 K, so that it is directly connected with the ferromagnetic ordering in the GaMnAs layer: Fig. 6 compares the temperature dependence of the spin-separation effect with other measurements characterizing the ferromagnetic properties of the '10 nm' sample. This demonstrates that the FM-induced spin polarization persists up to the Curie temperature. 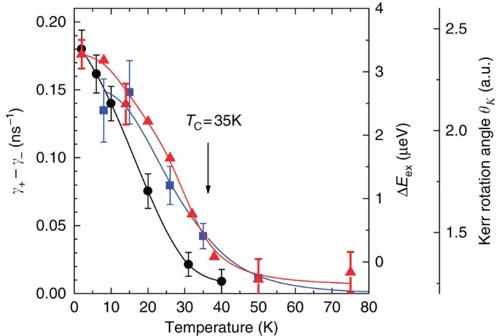Figure 6: Temperature dependence. Temperature dependence of difference between SDC ratesγ+−γ−atB=125 mT (circles), splitting ΔEex(T) evaluated from pump-probe Kerr rotation data (squares) and magnitude of Kerr rotation angleθK(T) atB=125 mT (triangles) for a photon energy 1.65 eV. The data are presented for the'10 nm' sample. A clear correlation between all three dependences is seen. Solid lines are guide to the eye. Figure 6: Temperature dependence. Temperature dependence of difference between SDC rates γ + − γ − at B =125 mT (circles), splitting Δ E ex ( T ) evaluated from pump-probe Kerr rotation data (squares) and magnitude of Kerr rotation angle θ K ( T ) at B =125 mT (triangles) for a photon energy 1.65 eV. The data are presented for the'10 nm' sample. A clear correlation between all three dependences is seen. Solid lines are guide to the eye. Full size image There are two main contributions to the FM-induced spin polarization of SC charge carriers [22] : the first one is the equilibrium spin polarization due to the thermal population of spin levels split by the exchange magnetic field of the FM. In this case, the FM layer acts as spin polarizer. The second one is the non-equilibrium polarization arising from the spin transfer through the FM–SC interface. Here the FM works as spin separator redistributing the spins spatially. The former mechanism is expected for FM/QW hybrids [13] , [14] , [15] , whereas the latter is demonstrated via the spin injection/reflection of free electrons at a FM–SC interface [3] , [5] , [6] , [20] , [24] . Here we show unambiguously that, in contrast to previous expectations [13] , [14] , [15] , the spin polarization in GaMnAs-based FM/QW hybrid is a non-equilibrium, dynamic one. Moreover, unlike [3] , [5] , [6] , [20] , [24] , the spin-separation effect considered here is due to the QW electrons and would take place even for the FM/QW hybrid embedded into insulating (that is, non-injection) structure. The results obtained on a FM–SC hybrid with a nanometer separation between the two layers open up the possibility of optical readout of the magnetization of the FM layer and control of the non-equilibrium QW electron spin, as, in particular, the excellent optical properties of the semiconductor layer are maintained. An important point here is that the FM-induced spin polarization persists up to the Curie temperature. This means that there are no other diminishing factors involved. A choice of materials involving a proper ferromagnetic layer might allow one to make the device operational at elevated temperatures. Experimental set-up and measurements In all measurements, the samples were placed in the variable temperature inset of an optical liquid-helium cryostat. Magnetic fields, up to 300 mT, were applied in Voigt (perpendicular to the growth axis) or Faraday (parallel to the growth axis) geometry, using an electromagnet. Photoluminescence For cw photoluminescence (PL) measurements the samples were optically excited by linearly/circularly polarized Ti-Sapphire or Kr + lasers (1.92 eV photon energy, laser spot diameter 0.1 mm). For time-resolved photoluminescence measurements, we used a mode-locked Ti-Sapphire laser-emitting pulses with a duration of 1 ps at 76 MHz rate and a single monochromator, equipped with a streak camera providing 20 ps time resolution. The photon energy was 1.44 eV, which corresponds to quasi-resonant below barrier excitation of the QW. All PL experiments were performed in back scattering geometry. Optical excitation and detection with either σ + or σ − polarization were selected by rotating a λ /4 plate in conjunction with a Glan-Thompson prism. Kerr rotation For magneto-optical Kerr rotation measurements, we applied a mode-locked Ti-Sapphire laser emitting pulses with a duration of 1 ps at 76 MHz. The rotation angle of the linearly polarized reflected probe pulse was homodyne, detected with a balanced photodiode and a lock-in amplifier. The magnetic field was applied along the growth axis [001] of the samples (Faraday geometry). To create optically oriented electrons, we used a pump-probe time-resolved Kerr rotation technique. Here we used the same Ti-Sapphire laser source split into pump and probe beams and tuned to the resonance with the QW exciton transition (photon energy 1.417 eV). Optical orientation of photo-excited carriers, by circularly polarized pump pulses, initiates a difference in the refraction indexes for σ + and σ − polarized light. As a result, linearly polarized probe pulses undergo a rotation of their polarization plane by an angle that is proportional to the [001]-projection of the photo-induced average spin. The pump-beam polarization was modulated between left and right circular with a photoelastic modulator operated at 40 kHz. The polarization rotation was homodyne detected in reflection using a polarization bridge in conjunction with balanced photodiodes. In addition, differential reflectivity measurements, where the intensity of the pump beam was modulated and the intensity of the reflected probe beam was homodyne detected, monitored the carrier kinetics in the studied structures with an overall time resolution of 2 ps. The latter provided complementary information on the lifetime of electron-hole pairs in the sample with 2 nm spacer thickness ( γ −1 =16 ps). How to cite this article: Korenev, V. L. et al . Dynamic spin polarization by orientation-dependent separation in a ferromagnet–semiconductor hybrid. Nat. Commun. 3:959 doi: 10.1038/ncomms1957 (2012).